Cellulose degradation and assimilation by the unicellular phototrophic eukaryoteChlamydomonas reinhardtii Plants convert sunlight to biomass, which is primarily composed of lignocellulose, the most abundant natural biopolymer and a potential feedstock for fuel and chemical production. Cellulose assimilation has so far only been described for heterotrophic organisms that rely on photosynthetically active primary producers of organic compounds. Among phototrophs, the unicellular green microalga Chlamydomonas reinhardtii is widely known as one of the best established model organisms. It occupies many habitats, including aquatic and soil ecosystems. This ubiquity underscores the versatile metabolic properties of this microorganism. Here we present yet another paradigm of adaptation for C. reinhardtii , highlighting its photoheterotrophic ability to utilize cellulose for growth in the absence of other carbon sources. When grown under CO 2 -limiting conditions in the light, secretion of endo-β-1,4-glucanases by the cell causes digestion of exogenous cellulose, followed by cellobiose uptake and assimilation. Phototrophic microbes like C. reinhardtii may thus serve as biocatalysts for cellulosic biofuel production. Cellulose is the most abundant natural product in the biosphere [1] , with plant cell walls representing the most important source, where it serves as a structural component [2] . During plant growth, the cell wall needs to be remodelled involving controlled degradation of cellulose by cellulolytic enzymes [2] . Many other organisms, preferring a heterotrophic lifestyle, also express cellulases. Cells of these organisms do not normally contain cellulose, but express a variety of cellulolytic enzymes rendering them capable of growth on cellulosic material as the sole carbon source [3] . Digestion of external cellulose requires the action of secreted cellulases, which belong to the glycoside hydrolase (GH) family of proteins and hydrolyse β-1,4 glycosidic bonds of the glucose polymer [4] . Cellulases can be grouped into endoglucanases, which cleave at random positions along the cellulose chain, thereby creating new chain ends, and exoglucanases that processively release oligosaccharides of defined length from the chain end [5] . The processive type of cellulase is crucial for efficient cellulose hydrolysis, and most of the characterized processive enzymes are exoglucanases, although endoglucanases of the processive type have been identified [6] . In the final step of cellulose utilization, small cellodextrins or cellobiose (CB) produced by endo-/exoglucanase activity have to be converted into glucose, and the conversion pathways differ between cellulolytic species. Enzymes involved in this process are β-glucosidases, cellodextrinases and cellodextrin phosphorylases, which can be localized intra- or extracellularly [3] . In contrast to heterotrophs, phototrophic microorganisms are not known to be capable of using cellulosic material as a carbon source for their growth. Among these photosynthetically active unicellular organisms, the eukaryotic green microalga Chlamydomonas reinhardtii is widely used for plant-related studies in the fields of molecular biology, systems biology and biotechnology [7] , [8] . This organism is arguably one of the best model systems available for biotechnology-driven light to biomass [9] , [10] and light to biofuel [11] production research. As a well-established genetic model system C. reinhardtii has the benefits of a fully sequenced genome [12] , existing transformation protocols, well-known biochemical pathways and culturing requirements. Importantly, this alga has yielded the highest rates of biomethane [13] and hydrogen production in eukaryotes to date [14] , [15] . Furthermore, C. reinhardtii combines plant, as well as animal features, and has retained many genes of the last common plant–animal ancestor, which were lost from the genomes of angiosperms (flowering plants) [12] . Another important difference between flowering plants and C. reinhardtii is its use of fermentative pathways characteristic for anaerobic chemotrophs, but not for oxygenic phototrophs, which can be explained by extended periods of anoxia experienced by this soil-dwelling photosynthetic microbe [16] . Like some other microalgae species, C. reinhardtii has the ability to grow both photoautotrophically with CO 2 as the sole carbon source or heterotrophically on acetate as an organic carbon source. In the case of C. reinhardtii , however, hexoses such as glucose cannot serve as the carbon source [17] , [18] . Its non-cellulosic cell wall [19] , [20] is solely composed of hydroxyproline-rich glycoproteins [21] . Although cellulose digestion as part of the cell wall remodelling process is not required in Chlamydomonas , the genome of this alga intriguingly contains genes encoding endo-β-1,4-glucanases and β-glucosidases ( Supplementary Table S1 ) known to be part of cellulolytic systems and GH family members potentially involved in hemicellulose degradation ( Supplementary Table S2 ). The potential existence of a complete enzymatic portfolio for cellulolysis and the non-cellulosic cell wall raised the question if, in contrast to the current understanding, this phototrophic organism also utilizes cellulose. As a result, we show in this work that C. reinhardtii is indeed able to use cellulosic material as an external carbon source under conditions of carbon dioxide limitation. Our new findings presented here, describe for the first time the ability of a photosynthetically active organism to utilize cellulosic material, which opens up the opportunity for future applications in biotechnologically driven approaches. C. reinhardtii secretes functional endo-β-1,4-glucanases In a first step we tested the ability of C. reinhardtii to degrade the water-soluble cellulose derivative carboxymethyl cellulose (CMC). Active digestion of CMC ( Fig. 1a ) by two different C. reinhardtii wild-type strains ( cc124 , cw10 ) within Congo red plate assays [22] caused a halo formation, suggesting CMCase secretion into the solid medium. In contrast, this phenotype could not be observed for the closely related microalga Chlorella kessleri , which uses a cellulosic cell wall [23] . Zymographic CMCase detection in culture supernatant samples ( Fig. 1b ) demonstrated a constant increase in the CMCase activity only during cultivation in the presence of CMC. This activity was exclusively found in the culture supernatant ( Fig. 1c ), and identification of two highly similar (64% identity) CMCases CrCel9B (UniProtKB A8JFG8) and CrCel9C (UniProtKB A8JFH1) within the secretome of this alga was achieved by affinity-based enrichment on microcrystalline cellulose (Avicel) in conjunction with mass spectrometric analysis ( Fig. 1d and Supplementary Table S3 ). Both proteins belong to GH family 9 (GHF9) with high homology to endo-β-1,4-glucanases from lower (for example, UniProtKB Q64I76) and higher (UniProtKB O77045) termites, as well as from earthworms (UniProtKB B9A7E3) [24] . Homology-based modelling [25] identified the GHF9 endo/exocellulase CelE4 from T. fusca [26] as a structural homologue of CrCel9B and endoglucanase AaCel9A from A. acidocaldarius [27] as a homologue of CrCel9C ( Supplementary Fig. S1 and Supplementary Table S1 ). In contrast to endogenous termite endoglucanases [28] , which typically contain only a catalytic GHF9 domain ( Supplementary Fig. S1 , NtEG) the algal enzymes possess an additional unknown type of module at either the carboxy (CrCel9B) or amino terminus (CrCel9C). Enrichment of the C. reinhardtii cellulases by purification on Avicel argues for a cellulose-binding function of the extra modules in CrCel9B/C, as efficient binding of GHF9 endoglucanases to microcrystalline cellulose requires binding modules in addition to the catalytic domain [29] . 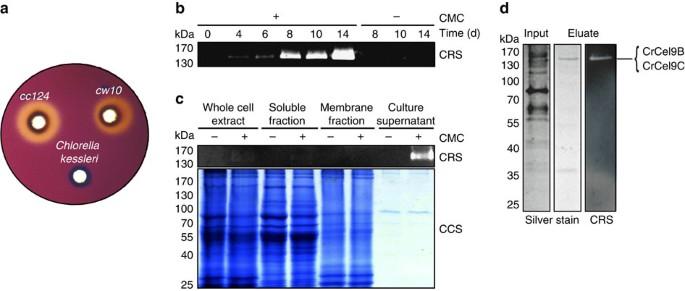Figure 1:C. reinhardtiicells secrete cellulolytic enzymes after media supplementation with carboxymethyl cellulose. (a) Congo red staining (CRS) of minimal media (MM) agar plates withC. reinhardtii(cc124;cw10) andChlorella kessleriwild-type colonies supplemented with 0.1% (w/v) carboxymethyl cellulose (CMC), 5 days after inoculation and growth under continuous illumination with 40 μmol m−2s−1. (b) Cellulolytic activity ofC. reinhardtii cc124wild-type cultures cultivated in MM with (+) or without (−) 0.1% (w/v) CMC, visualized by zymogram assays of the culture supernatant taken at the indicated time points (d, days of cultivation) of cultivation. (c) Localization of the CMCase activity by zymography (CRS) using subcellular fractions ofC. reinhardtiicells collected after 8 days of cultivation in CMC-containing MM (+) or CMC-free MM (−) and colloidal Coomassie staining (CCS) served as a loading control. (d) Identification of two secretedC. reinhardtiiCMCases by tandem mass spectrometry (MS/MS)de novosequencing after Avicel purification from a secretome sample (input) and zymographic (CRS) detection. Figure 1: C. reinhardtii cells secrete cellulolytic enzymes after media supplementation with carboxymethyl cellulose. ( a ) Congo red staining (CRS) of minimal media (MM) agar plates with C. reinhardtii ( cc124 ; cw10 ) and Chlorella kessleri wild-type colonies supplemented with 0.1% (w/v) carboxymethyl cellulose (CMC), 5 days after inoculation and growth under continuous illumination with 40 μmol m −2 s −1 . ( b ) Cellulolytic activity of C. reinhardtii cc124 wild-type cultures cultivated in MM with (+) or without (−) 0.1% (w/v) CMC, visualized by zymogram assays of the culture supernatant taken at the indicated time points ( d , days of cultivation) of cultivation. ( c ) Localization of the CMCase activity by zymography (CRS) using subcellular fractions of C. reinhardtii cells collected after 8 days of cultivation in CMC-containing MM (+) or CMC-free MM (−) and colloidal Coomassie staining (CCS) served as a loading control. ( d ) Identification of two secreted C. reinhardtii CMCases by tandem mass spectrometry (MS/MS) de novo sequencing after Avicel purification from a secretome sample (input) and zymographic (CRS) detection. Full size image Chlamydomonas cells utilize exogenous cellulosic material Secretion of active endoglucanases degrading water-soluble cellulose ( Fig. 1 ) indicated the existence of an enzymatic system for extracellular cellulose digestion in C. reinhardtii . Consequently, we analysed whether degradation products are used to fuel growth, which would imply the utilization of cellulosic material. Extracellular cellulose utilization by C. reinhardtii was demonstrated by growth experiments using high-salt minimal medium (MM) and air levels of carbon dioxide ( Fig. 2a ). Addition of CMC (MM+CMC) or filter paper (MM+FP) to Chlamydomonas wild-type cultures caused an increased exponential growth rate and a higher final cell density ( Fig. 2a ). Within this photoheterotrophic growth regime, it is not possible to discriminate between the contributions of photosynthesis and heterotrophic cellulose assimilation. We therefore analysed the growth-enhancing effect of cellulosic material in cultures of photosynthetic mutants from C. reinhardtii ( Fig. 2b ), which were supplemented with only a very low concentration of acetate (10% of the standard TAP (tris-acetate phosphate) medium [30] content), required for initiation of cell growth before an induction of cellulase expression. When growth of the cc4148 (FUD16) non-photoautotrophic mutant [31] in cellulose-containing and cellulose-free medium was compared, a biphasic curve resulted ( Fig. 2b ). Acetate assimilation in the initial phase ( Fig. 2b , right y axis, dotted lines, first 2 days) led to growth with comparable rates for all cultures, but an earlier stagnation of growth in the cellulose-free culture ( Fig. 2b , left y axis, black continuous curve) indicated assimilation of cellulose in the FP/CMC-containing cultures ( Fig. 2b , red and green continuous curves) after the medium was depleted of acetate ( Fig. 2b , right y axis, dotted lines, day 0 versus days 2–12), which takes only 2–3 days even if the standard acetate amount is used for cultivation [32] . It is important to note that all cultures grew at almost identical rates under acetate-replete conditions, so that differences in the assimilation rate of acetate can be excluded as the cause for the higher growth rate in the cellulose-containing cultures. Addition of cellulosic material to medium containing a lowered amount of acetate caused a delayed transition from the exponential to the stationary growth phase and increased the final cell density considerably (249±17% FP and 295±15% CMC versus 100% cellulose-free culture, values±(s.d.) with n =9). Similar results ( Fig. 2c , 156±5.85% (s.d./ n =6) with FP versus 100% without cellulose on day 6) were obtained with another photosynthetic mutant cc4147 ( FUD7 ) [33] . In addition to experiments carried out in MM containing a low amount of acetate, cellulose assimilation of photosynthetic mutant FUD16 was also analysed under conditions where cellulose was the sole organic carbon source present in the medium ( Fig. 2d ). Under these conditions, the photosynthetic mutant has to establish a cellulose-degrading environment without the aid of low acetate amounts in the initial phase of the growth experiment, which causes an extended lag-phase ( Fig. 2d , green curve, first 4 days). However, addition of cellulose ( Fig. 2d , MM+FP, green curve) resulted in growth of photosynthetic mutant FUD16 and caused a significantly higher final cell density (153±7.3% (s.d./ n =6) FP versus 100% MM). Chlamydomonas reinhardtii is therefore capable of heterotrophic cellulose assimilation. 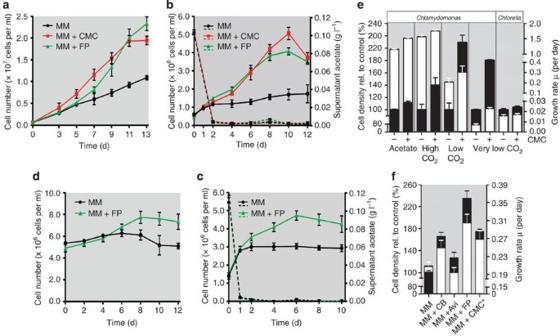Figure 2: Improved growth phenotype ofC. reinhardtiicell cultures after addition of cellulosic material. Error bars represent s.d. derived from three biological replicates, each including at least two technical replicates. (a–c) Growth analyses of (a) wild-typecc124, (b) the non-phototrophic mutantcc4148 (FUD16)and (c) the non-phototrophic mutantcc4147(FUD7), grown in MM without or with the addition of CMC (MM+CMC) or FP (MM+FP). For cultivation inbandc, MM were supplemented with 0.1 g l−1acetate. Acetate concentration (dotted lines) in the medium was monitored and plotted on the right y axis. (d) Mean cell densities of the non-phototrophic mutantFUD16cultivated in MM or in MM supplemented with FP (MM+FP). (e) Increases in final cell density (leftyaxis, black bars) and specific growth rate (rightyaxis, white bars) caused by cellulose addition (CMC; +) toC. reinhardtiiorChlorella kesslericultures. The growth-enhancing effect was determined in the presence of acetate or various carbon dioxide concentrations (high: 5% (v/v)/enriched air; low: ~0.04% (v/v)/air bubbling; very low: no bubbling) in MM. Final cell densities are given as relative changes (CMC-free cultivation set to 100%). (f) Final cell density (leftyaxis, black bars) and specific growth rate differences (rightyaxis, white bars) of air-bubbled cultures caused by addition of CB (MM+CB), Avicel (MM+Avi), FP (MM+FP) or CMC in the presence of antibiotic and fungicide (MM+CMC*). MM cultivation was set to 100%. Figure 2: Improved growth phenotype of C. reinhardtii cell cultures after addition of cellulosic material. Error bars represent s.d. derived from three biological replicates, each including at least two technical replicates. ( a – c ) Growth analyses of ( a ) wild-type cc124 , ( b ) the non-phototrophic mutant cc4148 (FUD16) and ( c ) the non-phototrophic mutant cc4147 ( FUD7 ), grown in MM without or with the addition of CMC (MM+CMC) or FP (MM+FP). For cultivation in b and c , MM were supplemented with 0.1 g l −1 acetate. Acetate concentration (dotted lines) in the medium was monitored and plotted on the right y axis. ( d ) Mean cell densities of the non-phototrophic mutant FUD16 cultivated in MM or in MM supplemented with FP (MM+FP). ( e ) Increases in final cell density (left y axis, black bars) and specific growth rate (right y axis, white bars) caused by cellulose addition (CMC; +) to C. reinhardtii or Chlorella kessleri cultures. The growth-enhancing effect was determined in the presence of acetate or various carbon dioxide concentrations (high: 5% (v/v)/enriched air; low: ~0.04% (v/v)/air bubbling; very low: no bubbling) in MM. Final cell densities are given as relative changes (CMC-free cultivation set to 100%). ( f ) Final cell density (left y axis, black bars) and specific growth rate differences (right y axis, white bars) of air-bubbled cultures caused by addition of CB (MM+CB), Avicel (MM+Avi), FP (MM+FP) or CMC in the presence of antibiotic and fungicide (MM+CMC*). MM cultivation was set to 100%. Full size image More detailed analyses of the growth-enhancing effect observed after addition of CMC ( Fig. 2a ) revealed that the growth-stimulating effect of CMC ( Fig. 2e , (+)) in comparison with CMC-free MM ( Fig. 2e , (−)) was inversely correlated to the availability of other carbon sources, such as carbon dioxide (high, low, very low CO 2 ) or acetate, indicating a special relevance of cellulose as an alternative carbon source ( Fig. 2e , right y axis, white bars). Under very low CO 2 conditions, where Chlamydomonas showed the largest specific growth rate increase caused by CMC addition, the growth rate of Chlorella kessleri was unaffected ( Fig. 2e , Chlorella , (−) versus (+)), which is explained by the fact that Chlorella does not secrete CMCases ( Fig. 1a ). The largest final cell density difference (209±11.9% (s.d.) with CMC versus 100% without CMC) between CMC-containing and CMC-free cultures was observed, when liquid cultures were bubbled with air, so that this condition was chosen for further analyses ( Fig. 2e , low CO 2 , left y axis, black bars). Importantly, addition of an antibiotic (25 μg ml −1 kasugamycin [34] ) together with a fungicide (5 μg ml −1 carbendacime [35] ) demonstrated that the growth-enhancing effect of CMC is not caused by a contaminant-assisted digestion process ( Fig. 2f , MM+CMC*). Growth rate and final cell density were even more increased when FP as a crystalline cellulose substrate was added ( Fig. 2f , MM+FP) and even the addition of Avicel as a very recalcitrant substrate improved growth, although to a smaller extent ( Fig. 2f , MM+Avi). Cellobiose, which is the final product of extracellular cellulose hydrolysis for many cellulolytic organisms, increased the final cell density of C. reinhardtii cultures when it was added as a culture supplement ( Fig. 2f , MM+CB). In conclusion, the addition of cellulosic compounds or of cellulose breakdown products, such as CB, clearly enhances the growth rate of this microalga. C. reinhardtii internalizes cellulose breakdown products Utilization of cellulose for cell growth requires enzymatic degradation to internalizable fragments (cellodextrins, CB). We therefore determined the specific cellulolytic activity found in crude C. reinhardtii supernatants on crystalline (FP, Avicel) and non-crystalline (CMC) substrates ( Table 1 ). In contrast to Chlorella , where no activity could be detected on either substrate, Chlamydomonas displayed activity on all analysed substrates with the highest activity on soluble cellulose ( Table 1 , CMC) and comparable activities for both crystalline substrates ( Table 1 , Avicel and FP). Not surprisingly, specific activities measured for C. reinhardtii were substantially lower than the activities previously reported for cellulolytic bacteria and fungi (87- to 218-fold CMC; 19- to 77-fold Avicel; 9- to 61-fold FP) [36] , [37] , [38] , [39] underscoring that this photosynthetic organism uses cellulose digestion as an extra mode of organic carbon acquisition and not as a main heterotrophic growth strategy, which would apply to saprophytes. Table 1 Hydrolytic activity of Chlamydomonas supernatant proteins on cellulosic substrates. Full size table In vitro hydrolysis of CMC using C. reinhardtii culture supernatants and subsequent analysis of digestion products revealed the formation of cellodextrins (cellotriose, cellotetraose and cellopentaose) as well as CB, only after cultivation in the presence of CMC ( Fig. 3a , CMC versus MM), and again no CMCase activity could be detected for Chlorella kessleri ( Fig. 3a , Chlorella ). As suggested by the increased growth rate ( Fig. 2f ) using FP and Avicel, even these crystalline substrates could be digested to CB ( Fig. 3a , FP and Avi). 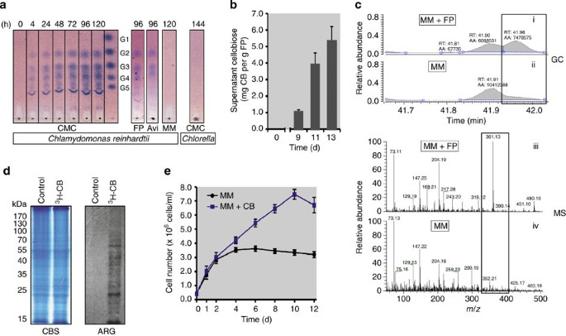Figure 3:In vitroandin vivoevidence for extracellular cellulose digestion and cellobiose uptake. Error bars (b,e) represent s.d. derived from four biological replicates each including two technical replicates. (a)In vitrodigestion of carboxymethyl cellulose (CMC), filter paper and Avicel (Avi) using culture supernatants ofChlamydomonasgrown with CMC or without supplements (MM).Chlorellawas grown in the presence of CMC and served as a control. Thin-layer chromatography was used to identify hydrolysis products after the indicated incubation times (h). Glucose (G1), cellobiose (G2), cellotriose (G3), cellotetraose (G4) and cellopentaose (G5) served as standards. (b) Detection and quantification of CB in culture supernatants ofC. reinhardtiicells grown in MM supplemented with crystalline cellulose (FP) by GC/MS. CB (mg CB × g−1FP) in the culture supernantant (y axis) was monitored during cultivation (xaxis; days (d) of cultivation). Error bars represent s.d. (c) Detection of CB in the intracellular metabolome ofC. reinhardtiicells grown in 0.1% (w/v) FP-containing MM (MM+FP). Gas chromatographic (GC) profiles (i, ii) and mass spectrometric (MS) analysis (iii, iv) of the eluate collected at a retention time of 41.96 min (black rectangle: i, ii). The peak at 361.13m/z(black rectangle, iii) represents the dominant mass of CB. Cell samples obtained by cultivation in FP-free media were used as a control (MM). (d) Import and assimilation of CB demonstrated by incubation ofC. reinhardtiiin the presence (3H-CB) or absence (control) of tritium-labelled CB. An autoradiogram of SDS–PAGE fractionated and blotted proteins (ARG) is shown together with a Coomassie (CBS) stain. (e) Growth analysis of a non-phototrophic mutant (cc4148 (FUD16)cultivated in the presence (blue curve) or absence (black curve, MM) of 3 mM CB (MM+CB). Cell densities (y axis) are given along with the time of cultivation (x axis) in days (d). Figure 3: In vitro and in vivo evidence for extracellular cellulose digestion and cellobiose uptake. Error bars ( b , e ) represent s.d. derived from four biological replicates each including two technical replicates. ( a ) In vitro digestion of carboxymethyl cellulose (CMC), filter paper and Avicel (Avi) using culture supernatants of Chlamydomonas grown with CMC or without supplements (MM). Chlorella was grown in the presence of CMC and served as a control. Thin-layer chromatography was used to identify hydrolysis products after the indicated incubation times (h). Glucose (G1), cellobiose (G2), cellotriose (G3), cellotetraose (G4) and cellopentaose (G5) served as standards. ( b ) Detection and quantification of CB in culture supernatants of C. reinhardtii cells grown in MM supplemented with crystalline cellulose (FP) by GC/MS. CB (mg CB × g −1 FP) in the culture supernantant (y axis) was monitored during cultivation ( x axis; days (d) of cultivation). Error bars represent s.d. ( c ) Detection of CB in the intracellular metabolome of C. reinhardtii cells grown in 0.1% (w/v) FP-containing MM (MM+FP). Gas chromatographic (GC) profiles (i, ii) and mass spectrometric (MS) analysis (iii, iv) of the eluate collected at a retention time of 41.96 min (black rectangle: i, ii). The peak at 361.13 m/z (black rectangle, iii) represents the dominant mass of CB. Cell samples obtained by cultivation in FP-free media were used as a control (MM). ( d ) Import and assimilation of CB demonstrated by incubation of C. reinhardtii in the presence ( 3 H-CB) or absence (control) of tritium-labelled CB. An autoradiogram of SDS–PAGE fractionated and blotted proteins (ARG) is shown together with a Coomassie (CBS) stain. ( e ) Growth analysis of a non-phototrophic mutant ( cc4148 (FUD16) cultivated in the presence (blue curve) or absence (black curve, MM) of 3 mM CB (MM+CB). Cell densities (y axis) are given along with the time of cultivation (x axis) in days (d). Full size image We next intended to demonstrate the conversion of crystalline cellulose (FP) to CB in situ . The supernatant of a culture growing in MM and supplemented with FP was subjected to gas chromatography/mass spectrometry (GC/MS) measurements ( Fig. 3b ) to detect and quantify CB. In good correlation with our growth analyses ( Fig. 2a ), which showed significant changes in the growth rate between FP-containing and cellulose-free cultures from day 9 onwards, CB could be detected on day 9 after the start of cultivation, and increased further ( Fig. 3b , grey bars, 5.3±0.9 mg CB per g of added FP on day 13). Apart from detection in the supernatant, CB could also be found inside the cells ( Fig. 3c , 0.4±0.07 mg CB per g of dried biomass). The detection of CB among the in vitro and in situ hydrolysis products, together with the finding that CB addition to MM improved the growth of C. reinhardtii ( Fig. 2f , MM+CB), suggested that CB is a cellulose breakdown product, which can be internalized by C. reinhardtii ( Fig. 3c ). Consequently, CB transport into C. reinhardtii cells and the ability to assimilate this disaccharide were examined. Addition of radiolabelled 3 H-CB to C. reinhardtii cultures resulted in the incorporation of radiolabel into proteins, demonstrating active uptake and further utilization of external CB ( Fig. 3d , ARG, 3 H-CB). The ability of C. reinhardtii to grow strictly heterotrophic on CB was further proven by growth analyses ( Fig. 3e ) using the non-phototrophic mutant cc4148 (FUD16) [31] , which were conducted in the same way as FP and CMC growth-enhancing effects were determined ( Fig. 2b ), except for the replacement of cellulose by CB. Again, a biphasic curve was observed with almost identical growth rates of CB-containing and CB-free cultures under acetate-replete conditions (until day 2 after the start of cultivation). After the second day of cultivation, the CB-containing culture showed an increased growth rate ( Fig. 3e , blue curve, MM+CB), resulting in a higher final cell density (220±6.7% for MM+CB versus MM set to 100% on day 10). The demonstrated ability to import CB might explain, why this green microalga does not possess a hexose uptake system [17] , [18] . So far, only a few CB transporters have been identified belonging to the major facilitator superfamily [40] or the ATP-binding cassette transporter family [41] , and members of both are encoded by the Chlamydomonas nuclear genome (for example, UniProtKB A8J114/A8ILE4). In vitro hydrolysis assays carried out with C. reinhardtii culture supernatants, as well as the general capability of CB uptake and assimilation, indicated that this alga degrades different cellulosic substrates and internalizes resulting fragments. In summary, we conclude that C. reinhardtii converts soluble and crystalline cellulose to CB, which can be transported into the algal cell and subsequently fed into metabolism, as indicated by tritium-labelling experiments. Sensing of exogenous cellulose induces cellulase expression Determination of mRNA steady-state levels concerning the identified GHF9 cellulase and β-glucosidase genes implies the existence of a substrate-induced signalling mechanism for the induction of cellulolytic activity ( Fig. 4 ). The amount of mRNAs encoding the cellulases identified in the culture supernatant (Fig. 1c ) showed a 2.3- ( CrCel9B ) or 3.5-fold ( CrCel9C ) increase in the presence of FP compared with cultivation in the absence of cellulose ( Fig. 4a ). Interestingly, mRNA expression of the third cellulase CrCel9D could only be detected when FP was added to the medium, demonstrating a more stringent substrate-dependent regulation of this gene ( Fig. 4b ). Common to all three cellulase genes was that supplementation of the medium with CB had a negligible effect on the mRNA amount ( Fig. 4a , MM+CB versus MM+FP). In contrast to this, mRNA expression of the two intracellularly located β-glucosidases CrBGl1/2 was increased after addition of both CB and FP, suggesting a direct correlation between substrate availability and expression induction ( Fig. 4c ). In summary, the data demonstrate an expression induction of the cellulolytic system including cellulases and β-glucosidases, if crystalline cellulose is present in the microenvironment of the algal cell. 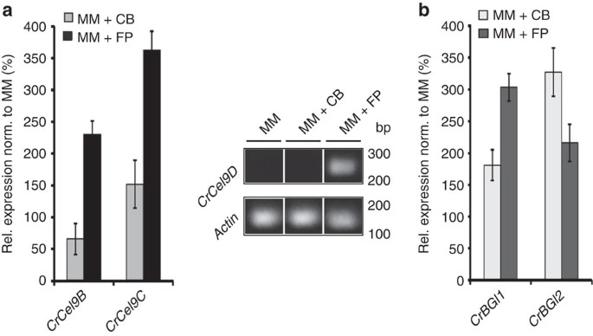Figure 4: Induction of cellulase expression by the addition of crystalline cellulose toC. reinhardtiicultures. mRNA expression analyses of the three cellulase genesCrCel9B/C/D(a) and the two β-glucosidase genesCrBGl1/2(b) were performed using RNA samples from cultures containing FP or CB. (a) Left panel: relative changes in theCrCel9B/CmRNA steady-state levels after addition of CB (MM+CB) or FP (MM+FP) to MM determined by quantitative RT–PCR (left panel). Growth in MM without supplements served as a reference condition (set to 100%). Error bars indicate the s.d. (n=8) of two biological replicates, including four technical replicates. Right panel: detection ofCrCel9Dandβ-actin(control) mRNAs by SYBR safe staining of gel-separated RT–PCR products. (b) Increases in the mRNA steady-state levels of the two β-glucosidase genesCrBGl1/2after addition of FP (MM+FP) or CB (MM+CB) to MM. Figure 4: Induction of cellulase expression by the addition of crystalline cellulose to C. reinhardtii cultures. mRNA expression analyses of the three cellulase genes CrCel9B/C/D ( a ) and the two β-glucosidase genes CrBGl1/2 ( b ) were performed using RNA samples from cultures containing FP or CB. ( a ) Left panel: relative changes in the CrCel9B/C mRNA steady-state levels after addition of CB (MM+CB) or FP (MM+FP) to MM determined by quantitative RT–PCR (left panel). Growth in MM without supplements served as a reference condition (set to 100%). Error bars indicate the s.d. ( n =8) of two biological replicates, including four technical replicates. Right panel: detection of CrCel9D and β-actin (control) mRNAs by SYBR safe staining of gel-separated RT–PCR products. ( b ) Increases in the mRNA steady-state levels of the two β-glucosidase genes CrBGl1/2 after addition of FP (MM+FP) or CB (MM+CB) to MM. Full size image The closed circle of reaction processes that includes the substrate-induced transcription of cellulases and β-glucosidases, secretion of expressed cellulases, digestion of cellulosic material to CB and the import of CB into the cell ( Fig. 5 ) is a perfect example for C. reinhardtii as a multifunctional ‘planimal’. In our current view, a cellulose digestive system is expressed if crystalline cellulose is provided as an inductor. Limited cellulose hydrolysis is often viewed as the trigger for an expression of the full array of enzymes implicated in cellulose utilization and requires a basal level of cellulases in the secretome under all conditions [3] , [42] . Our data demonstrate that CrCel9B and CrCel9C fulfil this function, and that CrCel9D is only recruited if the algal cell senses degradable material in its environment. Cellulolytic eukaryotes studied so far prefer a strictly heterotrophic lifestyle and evolved a sophisticated system employing a great number of different endo- and exoglucanases, as well as enzymes needed for lignocellulose digestion [3] . The Chlamydomonas system is simpler, which can be attributed to the fact that this mainly phototrophic organism does not completely rely on cellulose utilization, as can be stated for saprophytes. Cellulosic material rather represents an extra carbon source, which has a special relevance under conditions of carbon dioxide limitation. It is not surprising that this system employs cellulases belonging to GHF9, which is the most conserved family of cellulases [43] , comprising endo- as well as exoglucanases, and enzymes of the processive type [44] , [45] . The ability to degrade soluble (CMC) and crystalline (FP, Avicel) cellulosic substrates to small cellodextrines and CB allows the only conclusion, that the secretome of C. reinhardtii contains an endo-/exoglucanase system or at least one processive endoglucanase. In addition to the GHF9 enzymes, we could identify members of family 2, 3, 5, 27 and 28 ( Supplementary Table S2 ), which contain enzymes implicated in the degradation of hemicellulose or pectin. The partition of an exocellular polysaccharide digestion from an intracellular digestion to glucose can be explained as a strategy that ensures not only exclusive delivery of the end product to the cell metabolism but also prevents from unwanted glucose supply for competitors or potential pathogens in the microenvironment. With its non-cellulosic cell wall, this organism seems to be perfectly equipped for such a sophisticated strategy. It also provides an explanation why C. reinhardtii is able to occupy so many different habitats in nature. Most importantly, the ability of this microalga for substrate-mediated active secretion of endogenous cellulases fuels into recent biotechnologically driven efforts to engineer bioprocessing microbes such as S. cerevisiae and E. coli exactly with this phenotype to support cellulose digestion as a precondition for efficient production of biofuels [46] , [47] . Our new findings presented here will open up the opportunity of using a phototrophic microorganism for providing cellulases via secretion in suitable applications such as the sunlight-driven conversion of cellulosic paper waste material to biomass. 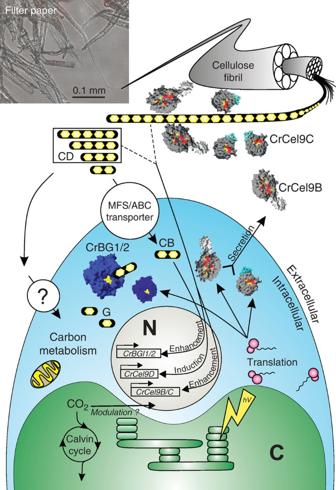Figure 5: Evidence for a regulatory mechanism inducing cellulolytic activity inC. reinhardtii. A model illustrating the potential mechanism inC. reinhardtiifor the use of cellulose as a carbon source for mixotrophic growth. CB, cellobiose; CD, cellodextrins; G, glucose; N, nucleus; C, chloroplast Figure 5: Evidence for a regulatory mechanism inducing cellulolytic activity in C. reinhardtii . A model illustrating the potential mechanism in C. reinhardtii for the use of cellulose as a carbon source for mixotrophic growth. CB, cellobiose; CD, cellodextrins; G, glucose; N, nucleus; C, chloroplast Full size image Strains and culture conditions Liquid cultures of Chlamydomonas reinhardtii wild-type strain cc124 [137c] and Chlorella kessleri (Parachlorella kessleri ; SAG 211-11h) were cultivated phototrophically in high-salt MM and mixotrophically in TAP, or by adding different carbon sources to MM under continuous white light (100 μmol photons m −2 s −1 ) with or without bubbling (air or carbon dioxide-enriched air 5% (v/v)) [30] . The non-phototrophic mutants cc4148 ( FUD16 ) [31] and cc4147 ( FUD7 ) [33] were cultivated in low light (50 μmol photons m −2 s −1 ) and air-bubbled MM containing only 10% of the acetate concentration (1.7 mM) used in TAP [30] (17 mM). The following carbon sources were used at a concentration of 0.1% (w/v): CB, CMC (Carl Roth, 3333.1), Avicel (VWR, 1.02331.0500) or Whatman filter paper (Carl Roth, CL64.1). To exclude the risk of bacterial or fungal contaminations, the cells were additionally cultivated with the addition of antibiotics (25 μg ml −1 kasugamycin) [34] and fungicides (5 μg ml −1 carbendacime) [35] . The increase in cell density was monitored by cell counts using a haemocytometer (Neubauer Improved). Specific growth rates μ were calculated for the exponential phase using the following equation, where N 2 represents the cell number per ml at t 2 and N 1 the respective number at t 1 : The acetate concentration in the medium was determined using Acetic Acid Kit (Boehringer Mannheim/R-Biopharm; Product Code 10148261035) according to the manufacturer’s instructions. Solid 0.1% (w/v) CMC–MM plates were prepared using 1.5% (w/v) Select Agar (Gibco BRL). For the detection of cellulolytic activity on agar plates, 1 × 10 7 algal cells were added into a 7-mm diameter well and grown for 5 days before Congo red staining. Sample preparation and SDS–polyacrylamide gel electrophoresis Algal cultures supplemented with antibiotic (25 μg ml −1 kasugamycin) and fungicide (5 μg ml −1 carbendacime) were grown for 8 days and centrifuged at 2,500 g for 5 min to separate cells and culture supernatant. Cells were washed three times with PBS buffer (137 mM NaCl, 2.7 mM KCl, 4.3 mM Na 2 HPO 4 , 1.4 mM KH 2 PO 4 , pH 7.4) and disrupted by sonication on ice. Cell lysates were centrifuged at 16,000 g for 5 min to separate the soluble and insoluble protein fraction. The culture supernatant was centrifuged three additional times at 10,000 g for 15 min and then directly used for analysis. Protein concentration was determined by the Lowry assay [48] . Avicel-enrichment of supernatant proteins was performed as follows: 450 ml culture supernatant was lyophilized and re-dissolved in 16 ml 300 mM phosphate buffer (pH 7). Subsequently, 4 ml of the supernatant concentrate were mixed with 0.25 ml of 50% (v/v) Avicel slurry (washed, autoclaved and equilibrated in 300 mM phosphate buffer) and incubated for 30 min at 37 °C. The samples were subsequently centrifuged for 2 min at 3,000 g and the Avicel pellet was washed four times with TBS (50 mM Tris pH 7.4, 150 mM NaCl) before elution with 250 μl non-reducing SDS–polyacrylamide gel electrophoresis (PAGE) sample buffer. Eluted fractions destined for SDS–PAGE analysis and silver staining were precipitated with chloroform/methanol as described by Wessel and Flügge [49] . Samples for zymography were not further concentrated. SDS–PAGE was performed in 10% polyacrylamide gels according to Laemmli [50] . Protein bands were detected by staining with either PageBlue Protein Staining Solution (Thermo Scientific; catalogue number: 24620) or by silver staining [51] , [52] . Zymograms For gel-based CMCase detection 0.1% (w/v), CMC was added to the resolving gel solution [53] . Upon completion of electrophoresis, gels were washed twice for 30 min with 2.5% (w/v) Triton X-100, and re-activation of the enzymes was achieved by incubation in activity buffer (50 mM Tris HCl pH 7.4, 100 mM NaCl, 5 mM CaCl 2 , 10 μM ZnCl 2 , 1% (v/v) Triton X-100, 0.1% NaN 3 ) for 24 h at 42 °C. Cellulolytic activities on agar plates or polyacrylamide gels were visualized by staining with 0.2% (w/v) Congo red solution for 15 min at room temperature and destaining in 1 M NaCl [22] . In vitro hydrolysis assay In vitro hydrolysis reactions were performed in 96-well flat-bottom plates (Sarstedt) corresponding to King et al. [54] . Cell-free supernatants of C. reinhardtii or Chlorella kessleri cultivated in air-bubbled MM (±CMC) containing antibiotics (25 μg ml −1 kasugamycin) and fungicides (5 μg ml −1 carbendacime) were used for the in vitro hydrolysis assay. Three different assay substrates with a concentration of 1% (w/v) were investigated: CMC, Avicel and FP. The hydrolysis reactions were incubated at 42 °C for 4–144 h. Negative controls of the supernatant (without substrate) and substrate in assay buffer (without supernatant) were used to exclude chemical hydrolysis unrelated to cellulase activity. Digestion products were analysed by thin-layer chromatography using Merck 60F 254 silica gel plates according to Zhang and Lynd [55] . Reducing sugar quantification The DNS (3,5-dinitrosalicylic acid) reducing sugar assay was performed in a 96-well microplate format according to King et al. [54] , and DNS reagent was prepared as previously described [56] , [57] . GC/MS analyses Metabolite extraction of lyophilized cell and supernatant samples as well as derivatization for GC/MS analysis were performed as described before [32] . Metabolite identification and quantification were verified with purified standards (Merck, Germany). CB uptake studies C. reinhardtii cells ( cc124 [137c] ) were dark-incubated for 24 h in TAP medium supplemented with 10 μCi [ 3 H]–CB (specific activity, 4 Ci mmol −1 ). Cultures without radiolabel served as controls. After incubation, cells were washed five times with TAP medium. To detect the incorporation of radiolabel into proteins, cells were lysed with SDS–PAGE sample buffer [50] and proteins precipitated according to Wessel and Flügge [49] . Re-solubilized proteins were then separated by SDS–PAGE, using 12% polyacrylamide gels according to Laemmli [50] , and blotted onto a nitrocellulose membrane. The dried membrane was subsequently incubated with Amersham Amplify Fluorographic Reagent (NAMP100, GE Healthcare) for 30 min before the detection of radioactivity using X-ray films (Hyperfilm MP, GE Healthcare). Protein loading was assessed by colloidal Coomassie blue staining. Trypsin digestion and mass spectrometry In-gel digestion with trypsin and mass spectrometry analysis was performed as described previously [58] . Real-time quantitative reverse-transcription PCR Real-time reverse transcription PCR (RT–PCR) was performed as described in a previous study [9] , using the SensiMix One-Step kit (Quantace) in conjunction with the DNA Engine Opticon system (Bio-Rad). Primer sequences are listed in Supplementary Table S4 . Ab initio modelling Ab initio modelling of the three-dimensional structure of the proteins was performed by applying I-TASSER (Centre for Computational Medicine and Bioinformatics University of Michigan, USA) to the amino acid sequences of CrCel9B and CrCel9C (UniProtKB A8JFG8 and A8JFH1) according to Roy et al. [25] The surface plots were calculated using the software DeepView-Swiss-PdbViewer [59] . How to cite this article: Blifernez-Klassen, O. et al. Cellulose degradation and assimilation by the unicellular phototrophic eukaryote Chlamydomonas reinhardtii . Nat. Commun. 3:1214 doi: 10.1038/ncomms2210 (2012).